Ndfip1 restricts mTORC1 signalling and glycolysis in regulatory T cells to prevent autoinflammatory disease Foxp3 + T regulatory (T reg ) cells suppress immune cell activation and establish normal immune homeostasis. How T reg cells maintain their identity is not completely understood. Here we show that Ndfip1, a coactivator of Nedd4-family E3 ubiquitin ligases, is required for T reg cell stability and function. Ndfip1 deletion in T reg cells results in autoinflammatory disease. Ndfip1-deficient T reg cells are highly proliferative and are more likely to lose Foxp3 expression to become IL-4-producing T H 2 effector cells. Proteomic analyses indicate altered metabolic signature of Ndfip1-deficient T reg cells and metabolic profiling reveals elevated glycolysis and increased mTORC1 signalling. Ndfip1 restricts T reg cell metabolism and IL-4 production via distinct mechanisms, as IL-4 deficiency does not prevent hyperproliferation or elevated mTORC1 signalling in Ndfip1-deficient T reg cells. Thus, Ndfip1 preserves T reg lineage stability and immune homeostasis by preventing the expansion of highly proliferative and metabolically active T reg cells and by preventing pathological secretion of IL-4 from T reg cells. Foxp3 + regulatory T (T reg ) cells suppress spontaneous immune cell activation and limit effector cell function, thereby preventing autoimmune and inflammatory disorders [1] , [2] . While generally stable, T reg lineage cells can have a high degree of instability in inflammatory settings. T reg cell instability is characterized by the loss of suppressive function, loss of Foxp3 protein or gain of pro-inflammatory cytokine production [3] , [4] . Defining pathways that help to establish and maintain Foxp3 expression, promote T reg cell suppressive function, prevent T reg cell production of pro-inflammatory cytokine and/or maintain T reg cell numbers will aid in the development of new T reg cell-based therapeutic applications. Appropriate regulation of cellular energetics and metabolism is important for T reg cell function and lineage stability [5] . Unlike effector T cells, which rely heavily on glycolysis, T reg cells rely on fatty acid oxidation for their energy needs [6] . Mechanistic target of rapamycin (mTOR) is a serine–threonine kinase that forms part of the mTORC1 and mTORC2 protein complexes and is a critical regulator of cellular metabolic processes. Both complexes can limit glycolysis in T reg cells thereby promoting lineage stability and suppressive functions [7] , [8] . Although metabolic state is clearly important for T reg maintenance and function, many factors that impact T reg cell metabolism remain unknown. Ubiquitylation is a fundamental post-translational modification affecting many aspects of T-cell differentiation and function [9] , [10] . Neural precursor cell expressed, developmentally downregulated 4 (Nedd4) family interacting protein 1 (Ndfip1) is a transmembrane protein that binds and activates Nedd4 family E3 ubiquitin ligases [11] . The highly conserved catalytic E3 ligases perform two functions in protein ubiquitylation: binding to the specific ubiquitylation target and catalysing the final transfer of ubiquitin. Ndfip1 activation of the Nedd4 E3 ligase Itch results in ubiquitylation and degradation of the transcription factor JunB, thereby limiting interleukin (IL)-4 cytokine production from T helper type 2 (T H 2) cells and T H 2-mediated inflammatory disease [12] , [13] . Ndfip1-deficient mice have decreased T reg cell numbers in the small bowel, a site of peripheral T reg generation, likely due to increased IL-4 signalling, which is inhibitory to T reg differentiation [14] . However, whether Ndfip1 also modulates T reg function after cells have committed to the T reg cell lineage has not been explored. Given that T reg -specific deletion of Itch results in a T H 2-biased autoinflammatory disease [15] , it seems plausible that Ndfip1 might be required to support Itch function in T reg cells. Here we show that Ndfip1 expression in T reg cells prevents spontaneous inflammation at several sites, such as the lungs and skin. Ndfip1 limits both the accumulation and proliferation of CD44 + effector T reg cells and prevents T reg cell production of IL-4. Consistent with increased proliferation and exposure to IL-4, T reg cells lacking Ndfip1 show increased conserved non-coding DNA sequence 2 (CNS2) methylation and are prone to losing Foxp3 expression in vivo. Increased T-cell proliferation is associated with increased mTORC1 signalling and high glycolytic activity, metabolic programmes that can fuel effector function in T reg cells and contribute to T reg lineage instability. Thus Ndfip1 maintains lineage identity in T reg cells and prevents these cells from aberrant acquisition of effector T-cell function. Ndfip1 is therefore a critical molecular sentinel that prevents autoinflammatory disease. T reg -specific loss of Ndfip1 results in inflammation Ndfip1 −/− mice develop a severe autoinflammatory disease by 6 weeks of age, resulting in death [12] , [16] . While thymic T reg output in Ndfip1-deficient mice is not altered [14] , T reg cell numbers are reduced at the sites of peripheral T reg induction [14] . Therefore, to test the role of Ndfip1 within committed T reg cells, we generated mice in which Ndfip1 is conditionally deleted in T reg cells using the Foxp3-Cre-YFP reporter mice [17] . We observed that Ndfip1 mRNA is induced upon stimulation of control Ndfip1 +/+ Foxp3- Cre-sorted YFP + T reg cells and that Ndfip1 message is effectively ablated in T reg cells from Ndfip1 fl/fl Foxp3- Cre male mice, which lack Ndfip1 in all T reg cells ( Fig. 1a ). 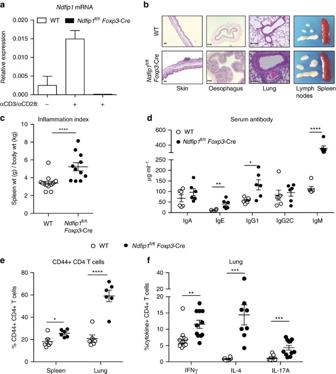Figure 1: Mice lacking Ndfip1 in their Tregcells develop inflammatory disease. (a)Ndfip1expression assessed by qPCR before (−) or after (+) αCD3/CD28 or PMA/ionomycin (P/I) stimulation of sorted YFP+Tregcells from WT andNdfip1fl/flFoxp3-Cre mice. A representative example ofNdfip1expression relative toActbafter αCD3/CD28 stimulation is shown. (b) Representative Haematoxylin and Eosin-stained histological sections of the skin, oesophagus and lung from genotypes as indicated are shown. Scale bars represent 100 μM. Far right image in panel is a representative image of the spleen and lymph nodes to illustrate size. (c) Inflammation index, calculated as a spleen weight/body weight for maleNdfip1+/+Foxp3-Cre (WT) andNdfip1fl/flFoxp3-Cre (cKO) mice at 9–16 weeks of age. (d) Levels of serum antibody isotypes as quantified by ELISA. (e,f) T cells from lung homogenates were analysed by flow cytometry for (e) the percentages of CD44+cells among CD4+cells and (f) the percentages of CD4+cells producing the indicated cytokines afterex vivo(P/I) stimulation.Pvalues determined by Student’st-test, with correction for unequal variances as appropriate. *P<0.05, **P<0.01, ***P<0.001, ****P<0.0001. Fora,c–f, bars indicate mean±s.e.m. Data inaare representative of four male animals of each genotype, 9–16 weeks, and forc–feach dot represents an individual male mouse aged between 9 and 16 weeks. All experiments were performed on at least two independent occasions. Figure 1: Mice lacking Ndfip1 in their T reg cells develop inflammatory disease. ( a ) Ndfip1 expression assessed by qPCR before (−) or after (+) αCD3/CD28 or PMA/ionomycin (P/I) stimulation of sorted YFP + T reg cells from WT and Ndfip1 fl/fl Foxp3- Cre mice. A representative example of Ndfip1 expression relative to Actb after αCD3/CD28 stimulation is shown. ( b ) Representative Haematoxylin and Eosin-stained histological sections of the skin, oesophagus and lung from genotypes as indicated are shown. Scale bars represent 100 μM. Far right image in panel is a representative image of the spleen and lymph nodes to illustrate size. ( c ) Inflammation index, calculated as a spleen weight/body weight for male Ndfip1 +/+ Foxp3- Cre (WT) and Ndfip1 fl/fl Foxp3- Cre (cKO) mice at 9–16 weeks of age. ( d ) Levels of serum antibody isotypes as quantified by ELISA. ( e , f ) T cells from lung homogenates were analysed by flow cytometry for ( e ) the percentages of CD44 + cells among CD4 + cells and ( f ) the percentages of CD4 + cells producing the indicated cytokines after ex vivo (P/I) stimulation. P values determined by Student’s t -test, with correction for unequal variances as appropriate. * P <0.05, ** P <0.01, *** P <0.001, **** P <0.0001. For a , c – f , bars indicate mean±s.e.m. Data in a are representative of four male animals of each genotype, 9–16 weeks, and for c – f each dot represents an individual male mouse aged between 9 and 16 weeks. All experiments were performed on at least two independent occasions. Full size image By 9–16 weeks of age, Ndfip1 fl/fl Foxp3- Cre male mice developed pronounced splenomegaly, lymphadenopathy and progressive dermatitis ( Fig. 1b ). Histologically, the skin, oesophagus and lung showed marked immune infiltration inflammation ( Fig. 1b ). Analysis of spleen weight-to-body weight ratios revealed that male Ndfip1 fl/fl Foxp3- Cre mice showed evidence of lymphoid expansion ( Fig. 1c ). To determine which immune responses were contributing to the observed inflammation, we examined serum immunoglobulin (Ig) levels. We found elevated levels of IgE and IgG1, indicative of type 2 inflammation, as well as elevated IgM ( Fig. 1d ). To determine the contribution of CD4 T cells to this pathology, we examined the spleen and lung of the mice and found increased activated phenotype (CD44 + ) CD4 T cells ( Fig. 1e ). CD4 T cells present in the lung of male Ndfip1 fl/fl Foxp3- Cre animals were more likely to express the effector cytokines interferon-γ (IFNγ), IL-4 and IL-17A upon ex vivo stimulation ( Fig. 1f ). These data suggested that Ndfip1 expression in T reg cells is required for suppression of tissue inflammation and pathology. Ndfip1 fl/fl Foxp3- Cre mice have more CD44 + eT reg cells The observed pathology could result from a loss of T reg cell numbers (as occurs with mice lacking Foxp3 [18] ) or T reg cell function (as is seen in T reg cell-specific CTLA4 deficiency [19] ). We therefore examined T reg percentages and numbers in the spleens and lung of Ndfip1 fl/fl Foxp3- Cre and controls. Surprisingly, T reg cell numbers were increased in Ndfip1 fl/fl Foxp3- Cre animals ( Fig. 2a–c ). Further, analysis of the T reg cell effector proteins—inducible T-cell costimulator (ICOS), programmed cell death-1 (PD-1) and glucocorticoid-induced TNFR-related protein (GITR)—revealed increased expression on T reg cells from Ndfip1 fl/fl Foxp3- Cre male mice compared to Cre + controls ( Fig. 2d ). We did not see marked changes in CD25 levels. Taken together, these data suggest that the immunopathology observed in Ndfip1 fl/fl Foxp3- Cre male mice is not due to decreased T reg numbers or loss of effector proteins known to support T reg function. 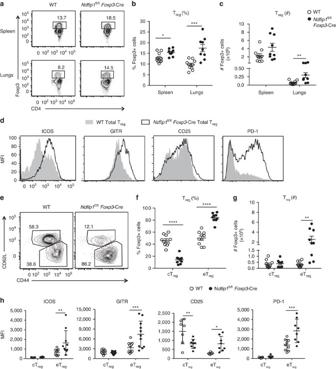Figure 2: Ndfip1-deficient eTregcells are increased in number and Tregcell surface expression. Tregcells from the spleens and lung (a–c) or lung (d–h) of 9–16-week-old male WT andNdfip1fl/flFoxp3-Cre mice were analysed by flow cytometry for numbers and surface markers. (a) Representative flow plots of Tregcells (previously gated as live CD3+CD4+cells) from the spleen and lung homogenates that were used to determine the percentages and total numbers. (b) Tregpercentages and (c) numbers compiled over multiple experiments. (d) Representative histograms of lung Tregcells (gated as ina) analysed for surface expression of ICOS, GITR, CD25 and PD-1. (e) Representative flow plots showing the gating of Tregcells that are effector (eTreg, CD44hiCD62Llo) or central (cTreg, CD62LhiCD44lo). This gating was used to determine the (f) percentages and (g) total numbers of these cells. (h) Quantification of mean fluorescence intensities (MFIs) of ICOS, GITR, CD25 and PD-1 on cTregcells and eTregcells.Pvalues were determined by Student’st-test, with correction for unequal variances as appropriate. *P<0.05, **P<0.01, ***P<0.001, ****P<0.0001. Each dot indicates data acquired from a single male mouse. Graphs with compiled data show mean±s.e.m. All experiments were performed on at least two independent occasions. Figure 2: Ndfip1-deficient eT reg cells are increased in number and T reg cell surface expression. T reg cells from the spleens and lung ( a – c ) or lung ( d – h ) of 9–16-week-old male WT and Ndfip1 fl/fl Foxp3- Cre mice were analysed by flow cytometry for numbers and surface markers. ( a ) Representative flow plots of T reg cells (previously gated as live CD3 + CD4 + cells) from the spleen and lung homogenates that were used to determine the percentages and total numbers. ( b ) T reg percentages and ( c ) numbers compiled over multiple experiments. ( d ) Representative histograms of lung T reg cells (gated as in a ) analysed for surface expression of ICOS, GITR, CD25 and PD-1. ( e ) Representative flow plots showing the gating of T reg cells that are effector (eT reg , CD44 hi CD62L lo ) or central (cT reg , CD62L hi CD44 lo ). This gating was used to determine the ( f ) percentages and ( g ) total numbers of these cells. ( h ) Quantification of mean fluorescence intensities (MFIs) of ICOS, GITR, CD25 and PD-1 on cT reg cells and eT reg cells. P values were determined by Student’s t -test, with correction for unequal variances as appropriate. * P <0.05, ** P <0.01, *** P <0.001, **** P <0.0001. Each dot indicates data acquired from a single male mouse. Graphs with compiled data show mean±s.e.m. All experiments were performed on at least two independent occasions. Full size image T reg cells can be quiescent or activated; these two subsets can be distinguished by the expression of CD44 and CD62L (ref. 20 ). Analysis of the lung of male Ndfip1 fl/fl Foxp3-Cre mice revealed an increase in frequency ( Fig. 2e,f ) and numbers ( Fig. 2g ) of Foxp3 + cells with an activated or ‘effector’ (eT reg ) phenotype (CD62L lo CD44 + ). In contrast, Ndfip1 fl/fl Foxp3- Cre and control mice contained equivalent numbers of cells with a quiescent or ‘central’ (cT reg ) phenotype (CD62L hi CD44 − ) ( Fig. 2g ). ICOS, PD-1 and GITR are more highly expressed on eT reg cells. In contrast, CD25 is particularly high on cT reg cells [20] . Thus the observed increase in surface expression of ICOS, PD-1 and GITR observed on total T reg cells from Ndfip1 fl/fl Foxp3- Cre animals could be due to an increased proportion of eT reg cells. To assess this, we examined the surface expression of ICOS, GITR, CD25 and PD-1 on the eT reg and cT reg populations. cT reg cells, as expected, had low levels of ICOS, GITR and PD-1, and loss of Ndfip1 did not alter this ( Fig. 2h ). However, cT reg cells from Ndfip1 fl/fl Foxp3- Cre mice had decreased levels of CD25. Strikingly, in addition to their increased frequency, eT reg cells from Ndfip1 fl/fl Foxp3- Cre mice showed higher levels of ICOS, GITR, CD25 and PD-1 compared to wild-type (WT) counterparts ( Fig. 2h ). cT reg cells are thymically derived and undergo peripheral conversion to eT reg cells under the instruction of T-cell receptor (TCR) stimulation and ICOS stimulation [20] . Therefore, observing increased frequency and number of eT reg cells could indicate either increased conversion of cT reg cells or expansion of eT reg cells. An increased cT reg conversion rate would be expected to decrease the numbers of cT reg cells, unless compensated for by thymic output. As there was no decrease in the peripheral numbers of cT reg cells in Ndfip1 fl/fl Foxp3- Cre male mice, we next examined thymic output utilizing mixed bone marrow chimera animals in which WT ( Ndfip1 +/+ Foxp3- Cre) and Ndfip1 fl/fl Foxp3- Cre T reg cells develop in the same environment to control for effects of inflammation. In control and mixed chimeras, total T reg thymic output was unchanged ( Supplementary Fig. 1a ). Furthermore, within the mixed chimeras there was no significant difference in the percentge of thymic T reg cells derived from Ndfip1-sufficient or -deficient cells relative to the observed reconstitution ratio of all thymic CD4 + T cells ( Supplementary Fig. 1b ). This suggests that the increase in eT reg , but not in cT reg , cell number in the periphery is not due to an altered rate of cT reg cell conversion to eT reg cells. Decreased suppressive function of T reg cells is known to lead to inflammation. Therefore, we examined T reg cell function . In vitro , Ndfip1-deficient and WT T reg cells suppressed proliferation of WT T conventional (T conv ) cells to the same degree ( Supplementary Fig. 1c,d ). We then examined T reg cell function in vivo using a model of T-cell transfer-induced colitis. Similar to our results from the in vitro assays, Ndfip1-deficient and WT T reg cells were equally able to prevent weight loss due to inflammation caused by cotransferred T conv cells ( Supplementary Fig. 1e ). These data support that the pathology observed in Ndfip1 fl/fl Foxp3- Cre mice is not due to a loss of T reg number or an overall loss of T reg cell-suppressive function. Ndfip1 limits T reg proliferation and levels of ICOS and GITR The expansion of CD44 + eT reg cells in male Ndfip1 fl/fl Foxp3- Cre animals in the absence of robust changes in cT reg cells suggested that Ndfip1 restricts eT reg cell numbers. Additionally, our data supported that Ndfip1 limits the expression of ICOS, GITR, CD25 and PD-1 on eT reg cells. However, both expansion and phenotype of eT reg cells could be altered in inflammatory environments, independent of an intrinsic role for Ndfip1. To distinguish between these possibilities, we examined Ndfip1 fl/fl Foxp3- Cre +/− female animals. These mice have mixtures of WT (YFP-Cre − ) and Ndfip1-deficient (YFP-Cre + ) Foxp3 + T reg cells, due to X chromosome inactivation, that can be distinguished by the expression of the YFP Cre reporter. Surprisingly, despite the presence of WT T reg cells, female Ndfip1 fl/fl Foxp3- Cre +/− mice had similar inflammatory burden, as defined by the ratio of spleen weight to body weight ( Supplementary Fig. 2a ) and contained equally high percentages of IFNγ-, IL-4- and IL-17A-expressing CD4 T cells, as the males ( Supplementary Fig. 2b ). Compared to male animals, which are uniformly sick beyond 16 weeks of age, female animals had lower incidence of skin dermatitis. Ndfip1 fl/fl Foxp3- Cre +/− mice contained increased numbers of total lung T reg cells compared to Ndfip1 +/+ Foxp3- Cre +/− counterparts ( Fig. 3a,b ). Similar to their male counterparts, female animals had total lung T reg cells that were skewed towards the eT reg phenotype ( Fig. 3c,d ). In control Ndfip1 +/+ Foxp3- Cre +/− female mice, Foxp3-Cre + (YFP + ) cells were outnumbered by Foxp3-Cre − (YFP − ) cells by almost 1:3, indicating an effect of Cre expression ( Fig. 3f ). Surprisingly, in Ndfip1 fl/fl Foxp3- Cre +/− females, this ratio was skewed towards YFP + cells, supporting an in vivo competitive advantage of Ndfip1-deficient T reg cells ( Fig. 3f ). 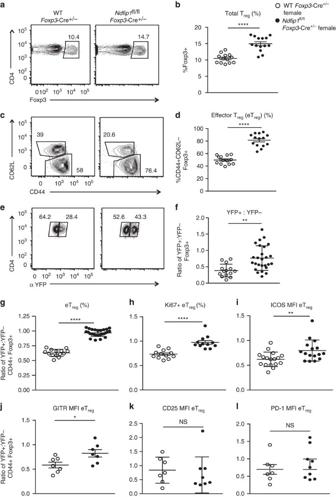Figure 3: FemaleNdfip1fl/flFoxp3-Cre+/−mice show similar Tregcell changes as males. (a–l) Lung homogenates, from 8- to 16-week-old hemizygous femaleNdfip1fl/flFoxp3-Cre+/−mice andNdfip1+/+Foxp3-Cre+/−controls, were analysedex vivoby flow cytometry. (a) Representative flow plots showing the gating of Tregcells (previously gated as live CD3+CD4+cells). This gating was used to determine the overall frequencies of Tregcells (b) in mice from the indicated genotypes. (c) Representative flow plots showing the gating of Tregcells fromathat are eTregor cTregcells. This gating was used to determine the (d) frequencies of eTregcells. (e) Representative flow plot of Tregcells as gated inaand analysed for frequencies of YFP+and YFP−cells. (f) Ratio of YFP+to YFP−Tregcells. (g,h) Percentages of (g) eTregcells or (h) Ki-67+eTregcells, shown as a ratio of YFP+:YFP−cells within each mouse to normalize for a Cre effect. (i–l) mean fluorescence intensity (MFI) of (i) ICOS, (j) GITR, (k) CD25 and (l) PD-1 expression on eTregcells, again shown as a ratio of YFP+:YFP−.Pvalues determined by Student’st-test, with correction for unequal variances as appropriate. *P<0.05, **P<0.01, ***P<0.001, ****P<0.0001. Each dot shows data acquired from a single female mouse. Graphs show mean±s.e.m. All experiments were performed on at least two independent occasions. Figure 3: Female Ndfip1 fl/fl Foxp3- Cre +/− mice show similar T reg cell changes as males. ( a – l ) Lung homogenates, from 8- to 16-week-old hemizygous female Ndfip1 fl/fl Foxp3- Cre +/− mice and Ndfip1 +/+ Foxp3- Cre +/− controls, were analysed ex vivo by flow cytometry. ( a ) Representative flow plots showing the gating of T reg cells (previously gated as live CD3 + CD4 + cells). This gating was used to determine the overall frequencies of T reg cells ( b ) in mice from the indicated genotypes. ( c ) Representative flow plots showing the gating of T reg cells from a that are eT reg or cT reg cells. This gating was used to determine the ( d ) frequencies of eT reg cells. ( e ) Representative flow plot of T reg cells as gated in a and analysed for frequencies of YFP + and YFP − cells. ( f ) Ratio of YFP + to YFP − T reg cells. ( g , h ) Percentages of ( g ) eT reg cells or ( h ) Ki-67 + eT reg cells, shown as a ratio of YFP + :YFP − cells within each mouse to normalize for a Cre effect. ( i – l ) mean fluorescence intensity (MFI) of ( i ) ICOS, ( j ) GITR, ( k ) CD25 and ( l ) PD-1 expression on eT reg cells, again shown as a ratio of YFP + :YFP − . P values determined by Student’s t -test, with correction for unequal variances as appropriate. * P <0.05, ** P <0.01, *** P <0.001, **** P <0.0001. Each dot shows data acquired from a single female mouse. Graphs show mean±s.e.m. All experiments were performed on at least two independent occasions. Full size image To identify intrinsic effects of Ndfip1 deficiency on T reg cells, in each female animal, for each parameter examined, we first determined the ratio of the value for YFP + -to-YFP − T reg cells to normalize for an effect of Cre. Then we compared this ratio between Ndfip1 fl/fl Foxp3- Cre +/− and Ndfip1 +/+ Foxp3- Cre +/− animals. Our analysis revealed that Ndfip1-deficient T reg cells were significantly more likely to display an eT reg phenotype (CD44 + CD62L lo ) ( Fig. 3g ). Furthermore, expression of the proliferative marker Ki67 ( Fig. 3h ) was increased in Ndfip1-deficient eT reg cells. eT reg cells lacking Ndfip1 also had significantly higher levels of ICOS ( Fig. 3i ) and GITR ( Fig. 3j ). Thus Ndfip1 restricts eT reg numbers by limiting their proliferation and their expression of ICOS and GITR. However, levels of CD25 and PD-1 were similar to controls ( Fig. 3k,l ), suggesting that these markers were not directly affected by the loss of Ndfip1 in T reg cells. The expression of activation markers on T reg cells is known to increase under inflammatory settings [20] . To determine how inflammatory conditions could influence control T reg cells, we looked at the expression of surface markers on CD44 + YFP − T reg cells from the Ndfip1 +/+ Foxp3- Cre +/− females or from the inflamed environment in Ndfip1 fl/fl Foxp3- Cre +/− female mice. CD44 + YFP − T reg cells from Ndfip1 fl/fl Foxp3- Cre +/− mice showed increased expression of ICOS, GITR, CD25 and PD-1 ( Supplementary Fig. 2c–f ). Taken together with the data in Figs 2 and 3 , this supports that the changes in CD25 and PD-1 expression in male Ndfip1 fl/fl Foxp3- Cre mice are secondary to inflammation and that while inflammation can increase levels of ICOS and GITR, Ndfip1 is also an intrinsic regulator of ICOS and GITR on T reg cells ( Supplementary Fig. 2g ). To further address whether the changes observed in the Ndfip1-deficient T reg cells were driven by inflammation, we looked in neonatal mice before the onset of overt inflammation. In 13-day-old female neonates, we found no differences between Ndfip1 fl/fl Foxp3- Cre +/− and Ndfip1 +/+ Foxp3- Cre +/− animals in spleen weight ( Supplementary Fig. 3a ), inflammation index ( Supplementary Fig. 3b ), total lung Foxp3 + T reg cell number or cytokine-producing CD4 T cells ( Supplementary Fig. 3c,d ). However, lungs from Ndfip1 fl/fl Foxp3-Cre +/− female mice contained greater frequencies of YFP + T reg cells ( Supplementary Fig. 3e ) and greater frequencies of eT reg cells ( Supplementary Fig. 3f ). Further, these eT reg cells showed higher expression of ICOS and GITR ( Supplementary Fig. 3g,h ). This further supports that Ndfip1 limits eT reg cell frequency and expression of ICOS and GITR in an intrinsic manner. Ndfip1 limits IL-4 production by T reg cells Our data indicate that Ndfip1 limits eT reg cell expression of ICOS and GITR and restricts eT reg cell proliferation. However, it remained unclear why Ndfip1 fl/fl Foxp3- Cre +/− females developed inflammation, when approximately half of the T reg cells in these mice are Ndfip1 sufficient. This suggested a pathological gain of function in Ndfip1-deficient T reg cells. We thus investigated whether Ndfip1-deficient T reg cells could contribute to the pool of cytokine-producing cells in the lung of Ndfip1 fl/fl Foxp3- Cre male mice shown in Fig. 1 . Effector cytokine production by WT T reg cells is relatively rare but has been described under inflammatory [21] or lymphopenic settings [22] , [23] . Strikingly, while WT T reg cells did not produce any IL-4 upon ex vivo stimulation, Ndfip1-deficient T reg cells could produce IL-4, and this was detectable at both the protein ( Fig. 4a,b ) and mRNA levels ( Fig. 4c ). Ndfip1-deficient T reg cells were also more likely to produce IL-10, IFNγ and IL-17A relative to WT controls. To determine whether the cytokine production was due to the loss of Ndfip1 or tied to the inflammatory environment, we generated mixed bone marrow chimeras. Consistent with our data from the female mice, these mixed chimeras developed dermatitis 8 weeks after reconstitution. Upon restimulation of lung homogenate, CD45.1 + WT Foxp3 + cells did not produce any IL-4 while CD45.2 + Ndfip1-deficient Foxp3 + cells in the same host could produce IL-4 ( Fig. 4d,e ), supporting an intrinsic role for Ndfip1 in limiting IL-4 production from T reg cells. Surprisingly, when we analysed the Foxp3 − T conv cells, we found a significant population of CD45.2 + cells that also expressed IL-4 ( Fig. 4f,g ), raising the possibility that the IL-4-producing population originated from Ndfip1 fl/fl Foxp3-Cre T reg cells that had lost Foxp3. 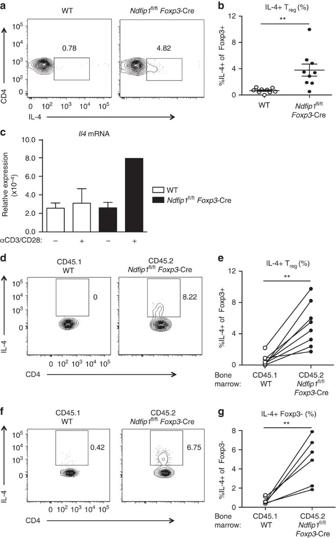Figure 4: Ndfip1-deficient Tregcells make IL-4. (a,b) Lung homogenates from WT andNdfip1fl/flFoxp3-Cre male mice aged 9–16 weeks were stimulatedex vivowith P/I and analysed for IL-4 production by flow cytometry. (a) Representative flow plots of Tregcells (Foxp3+CD3+CD4+) producing IL-4. (b) Compiled percentages of IL-4-producing Tregcells. (c) qPCR analysis ofIl4from sorted YFP+Tregcells from WT andNdfip1fl/flFoxp3-Cre male mice. Cells were unstimulated (−) or stimulated (+) with αCD3/CD28.Il4mRNA is shown relative toActb. (d–g) Lung homogenates from mixed chimeras were stimulatedex vivowith P/I and analysed for IL-4 production by flow cytometry. (d) Representative flow plots showing IL-4 production from Tregcells from WT (gated on CD45.1) orNdfip1fl/flFoxp3-Cre (gated on CD45.2) cells from the same recipient. (e) Graphs showing the percentages of IL-4+Tregcells from CD45.1 and CD45.2 cells in each chimera; cells from the same recipient are connected by a line. (f) Representative flow plots showing IL-4 production from Tconvcells from the same chimeras. (g) Graphs showing the percentages of IL-4+Tconvcells as pere. All experiments were performed on at least two independent occasions. Graphs show mean±s.e.m. Mixed bone marrow chimeras were generated and analysed in two separate experiments using male donors.Pvalues were determined by Student’st-test forb,cor pairedT-test. *P<0.05, **P<0.01. Figure 4: Ndfip1-deficient T reg cells make IL-4. ( a , b ) Lung homogenates from WT and Ndfip1 fl/fl Foxp3- Cre male mice aged 9–16 weeks were stimulated ex vivo with P/I and analysed for IL-4 production by flow cytometry. ( a ) Representative flow plots of T reg cells (Foxp3 + CD3 + CD4 + ) producing IL-4. ( b ) Compiled percentages of IL-4-producing T reg cells. ( c ) qPCR analysis of Il4 from sorted YFP + T reg cells from WT and Ndfip1 fl/fl Foxp3- Cre male mice. Cells were unstimulated (−) or stimulated (+) with αCD3/CD28. Il4 mRNA is shown relative to Actb . ( d – g ) Lung homogenates from mixed chimeras were stimulated ex vivo with P/I and analysed for IL-4 production by flow cytometry. ( d ) Representative flow plots showing IL-4 production from T reg cells from WT (gated on CD45.1) or Ndfip1 fl/fl Foxp3- Cre (gated on CD45.2) cells from the same recipient. ( e ) Graphs showing the percentages of IL-4 + T reg cells from CD45.1 and CD45.2 cells in each chimera; cells from the same recipient are connected by a line. ( f ) Representative flow plots showing IL-4 production from T conv cells from the same chimeras. ( g ) Graphs showing the percentages of IL-4 + T conv cells as per e . All experiments were performed on at least two independent occasions. Graphs show mean±s.e.m. Mixed bone marrow chimeras were generated and analysed in two separate experiments using male donors. P values were determined by Student’s t -test for b , c or paired T -test. * P <0.05, ** P <0.01. Full size image Ndfip1-deficient T reg cells lose Foxp3 expression Given the IL-4 production by Ndfip1-deficient T reg cells and their increased proliferative capacity, we posited that these cells would be likely to become methylated at their Foxp3 locus and become unstable. IL-4 receptor signalling in T reg cells, via signal transducer and activator of transcription factor 6 (STAT6), results in the methylation of the CNS2 region of the Foxp3 locus and repression of Foxp3 gene expression [24] . Therefore, we compared the methylation at 12 Cytosine-phosphate-guanine (CpG) islands in the Foxp3 CNS2 region in Ndfip1-sufficient and -deficient T reg cells, as well as WT T conv cells. As expected, the CNS2 CpG motifs were predominantly methylated in T conv cells ( Supplementary Fig. 4a ) [24] . Both WT and Ndfip1-deficient T reg cells had unmethylated CpG motifs in their Foxp3 promoter regions ( Supplementary Fig. 4b ), consistent with their expression of Foxp3 mRNA ( Supplementary Fig. 4c ). However, in Ndfip1 fl/fl Foxp3- Cre T reg cells, there was an increase in methylation at the 12 examined CNS2 CpG sites, compared to WT T reg cells, which remained unmethylated at these sites ( Fig. 5a,b ). 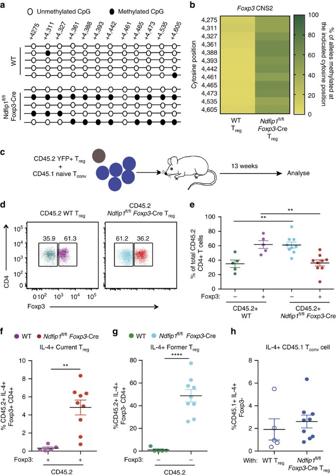Figure 5: Ndfip1-deficient Tregcells haveFoxp3locus instability and lose Foxp3in vivo. (a,b) YFP+eTregcells were sorted from 9- to 12-week-old WT orNdfip1fl/flFoxp3-Cre male mice and assessed for CNS2 methylation using bisulfite sequencing. (a) Representative data of methylation at theFoxp3CNS2 locus in Tregcells from the two genotypes. (b) Quantification of methylation at 12 CpG islands in theFoxp3CNS2 locus. Data shown are compiled from three mice of each genotype. Data are the percentage of alleles methylated at each position. (c–h) YFP+Tregcells from CD45.2+WT orNdfip1fl/flFoxp3-Cre mice were mixed 1:5 with CD45.1+WT naive Tconvcells and transferred toRag1−/−recipients. Cells from lung homogenates were analysed for Foxp3 and IL-4 expression using flow cytometry 13 weeks after transfer. (d) A representative flow plot showing CD45.2+WT andNdfip1fl/flFoxp3-Cre cells that were analysed for the expression of Foxp3. (e) Compiled data from multiple mice analysed as ind. (f) Percentages of IL-4-producing cells that remained Foxp3+(current Tregcells ) and (g) that had become Foxp3−following transfer (former Tregcells ). (h) Percentages of IL-4-producing CD45.1 Tconvcells. All experiments were performed on at least two separate occasions. Each dot represents cells from an individual mouse.Pvalues were calculated by one-way ANOVA. *P<0.05, **P<0.01, ***P<0.001, ****P<0.0001. Graphs show mean±s.e.m. Figure 5: Ndfip1-deficient T reg cells have Foxp3 locus instability and lose Foxp3 in vivo . ( a , b ) YFP + eT reg cells were sorted from 9- to 12-week-old WT or Ndfip1 fl/fl Foxp3- Cre male mice and assessed for CNS2 methylation using bisulfite sequencing. ( a ) Representative data of methylation at the Foxp3 CNS2 locus in T reg cells from the two genotypes. ( b ) Quantification of methylation at 12 CpG islands in the Foxp3 CNS2 locus. Data shown are compiled from three mice of each genotype. Data are the percentage of alleles methylated at each position. ( c – h ) YFP + T reg cells from CD45.2 + WT or Ndfip1 fl/fl Foxp3- Cre mice were mixed 1:5 with CD45.1 + WT naive T conv cells and transferred to Rag1 −/− recipients. Cells from lung homogenates were analysed for Foxp3 and IL-4 expression using flow cytometry 13 weeks after transfer. ( d ) A representative flow plot showing CD45.2 + WT and Ndfip1 fl/fl Foxp3- Cre cells that were analysed for the expression of Foxp3. ( e ) Compiled data from multiple mice analysed as in d . ( f ) Percentages of IL-4-producing cells that remained Foxp3 + (current T reg cells ) and ( g ) that had become Foxp3 − following transfer (former T reg cells ). ( h ) Percentages of IL-4-producing CD45.1 T conv cells. All experiments were performed on at least two separate occasions. Each dot represents cells from an individual mouse. P values were calculated by one-way ANOVA. * P <0.05, ** P <0.01, *** P <0.001, **** P <0.0001. Graphs show mean±s.e.m. Full size image These data suggested that Ndfip1 deficiency, via concomitant expression of IL-4, negatively impacts lineage stability of T reg cells. To test whether Ndfip1-sufficient and -deficient T reg cells have differential responses to destabilizing cytokines, we cultured Ndfip1-sufficient and -deficient Foxp3 + cells in stabilizing (IL-2) or destabilizing (IL-4 plus anti-IL-2) conditions and analysed Foxp3 protein expression as a surrogate for lineage stability. We found that Ndfip1-deficient T reg cells were equally stabilized by IL-2 and destabilized by IL-4 compared to their Ndfip1-sufficient counterparts ( Supplementary Fig. 4d,e ). Thus Ndfip1-deficient T reg cells are not uniquely sensitive to the destabilizing effects of IL-4; in vivo , however, Ndfip1-deficient IL-4 producing T reg cells are more likely to encounter destabilizing cytokine milieus. To test T reg lineage stability in vivo , we sorted WT or Ndfip1-deficient CD45.2 + YFP + T reg cells and cotransferred them with sorted naive CD45.1 + WT T conv cells into Rag1 −/− hosts ( Fig. 5c ). As we had previously observed ( Supplementary Fig. 1e ), mice receiving either Ndfip1-deficient or -sufficient T reg cells did not develop colitis ( Supplementary Fig. 5a ). At harvest, we determined the frequencies of CD45.2 + cells that were still Foxp3 + (current T reg cells) or that had lost Foxp3 (former T reg cells). In mice that received WT T reg cells, on average, 30% had lost Foxp3, similar to previous reports by other groups [8] , [22] . Strikingly, in mice that had received Ndfip1-deficient T reg cells, 60% on average had lost expression of Foxp3 ( Fig. 5d,e ). These Foxp3 − CD45.2 + cells could represent Ndfip1-deficient T reg cells that had lost Foxp3 expression in vivo or a very proliferative T conv cell contamination from cell sorting. If the Foxp3 − cells represented former T reg cells, they would lack Ndfip1 mRNA, due to excision following the expression of Foxp3-Cre. Contaminating T conv cells, on the other hand, would continue to express Ndfip1 . We sorted current T reg cells, former T reg cells and T conv cells and stimulated to induce the Ndfip1 mRNA expression. We found that the WT T conv cells expressed Ndfip1 mRNA, while neither the Ndfip1 fl/fl Foxp3-Cre + current T reg cells nor former T reg cells expressed detectable levels of Ndfip1 mRNA ( Supplementary Fig. 5b ). Thus T reg cells lacking Ndfip1 were more likely to lose Foxp3 expression than their WT counterparts. Current ( Fig. 5f ) and former ( Fig. 5g ) T reg cells lacking Ndfip1 produced IL-4, while current and former WT T reg cells did not. Importantly, none of the WT T conv cells produced IL-4 ( Fig. 5h ). This was not true for all cytokines since WT and Ndfip1-deficient cells were equally likely to make IFNγ regardless of whether they were T reg cells ( Supplementary Fig. 5c,d ) or cotransferred T conv cells ( Supplementary Fig. 5e ). Additionally, compared to WT T reg cells, Ndfip1-deficient T reg cells expanded to greater numbers in vivo ( Supplementary Fig. 5f,g ) suggesting an advantage in proliferation and/or survival of both current and former Ndfip1-deficient T reg cells. However, at steady state, it is likely that only a small percentage of Ndfip1 fl/fl Foxp3-Cre + T reg cells are actively losing their Foxp3 at any point of time. In support of this, Ndfip1-deficient total T reg cells, eT reg cells and cT reg cells from female animals do not show a decrease in Foxp3 mean fluorescence intensity at steady state ( Supplementary Fig. 6 ). In summary, in a setting where T reg cells are pushed to undergo lymphopenia-induced proliferation, Ndfip1-deficient T reg cells have an advantage in growth and expansion, which leads to a large increase in total numbers of Ndfip1-deficient current and and former T reg cells. Since the majority of Ndfip1-deficient former T reg cells ( ∼ 50%) produce IL-4, this may explain the dramatic loss of Foxp3 observed in vivo . IL-4 is dispensable for Ndfip1-deficient eT reg expansion To assess whether IL-4 is required for the phenotypic changes in T reg cells lacking Ndfip1, we examined T reg cells in mice that lack both Ndfip1 and IL-4 ( Ndfip1 IL-4 double knockout or DKO mice) [25] . These animals do not show the overt signs of inflammation such as dermatitis [25] , [26] observed in age-matched Ndfip1 fl/fl Foxp3- Cre animals. We observed increased frequencies of T reg cells ( Supplementary Fig. 7a,b ) compared to IL-4-deficient controls. The Ndfip1-deficient T reg cells that lacked IL-4 were more proliferative than controls, as determined by Ki67 ( Supplementary Fig. 7c ). Similar to the Ndfip1 fl/fl Foxp3- Cre mice, T reg cells in the Ndfip1 IL-4 DKO mice were predominantly eT reg cells ( Supplementary Fig. 7d,e ). Additionally, the Ndfip1- and IL-4-deficient eT reg cells expressed higher levels of Ki67 ( Supplementary Fig. 7f ) and ICOS ( Supplementary Fig. 7g ) relative to control eT reg cells. Thus, while IL-4 from current and former T reg cells likely contributes to the inflammation observed in Ndfip1 fl/fl Foxp3- Cre mice, increased T reg cell activation, proliferation and ICOS expression are not due solely to IL-4 signalling. Thus IL-4 is insufficient to explain the increased fitness of Ndfip1-deficient T reg cells. Ndfip1-deficient eT reg cells have altered metabolic activity To identify molecular pathways underlying the increased proliferation and altered eT reg cell phenotype of Ndfip1 deficient T reg cells, we used label-free quantitative proteomics to compare WT and Ndfip1-deficient cT reg and eT reg cells. We sorted YFP + eT reg and cT reg cells from young WT or Ndfip1 fl/fl Foxp3- Cre male mice, subjected these cells to liquid chromatography-tandem mass spectrometry (LC-MS/MS) analysis and quantified protein abundance using intensity-based absolute quantification [27] , [28] , [29] ( Fig. 6a ). We achieved good reproducibility of identified proteins across three experiments, pooling two to three mice of each genotype per experiment ( Fig. 6b ). Comparing proteins identified in control eT reg and cT reg proteomes, our data fit well with what has been published previously on proteins unique to each subtype. Namely, among proteins that were significantly more abundant in cT reg than eT reg proteomes or that were found exclusively in cT reg proteomes, defined here as having a cT reg ‘bias’, we identified CD62L and Bcl2 (ref. 20 ) ( Fig. 6c , Supplementary Data 1 ). Proteins that were increased in, or biased toward, the eT reg proteome included CD44 and several proteins associated with eT reg cells, such as Integrin alpha E/itgae (CD103) [30] ( Fig. 6c , Supplementary Data 1 ). 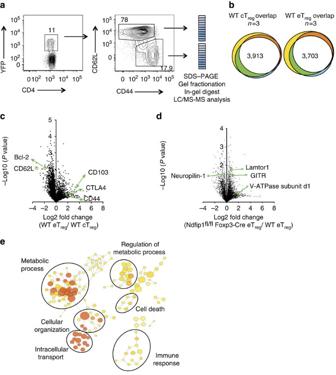Figure 6:Ndfip1fl/flFoxp3-Cre eTregcells have altered metabolic whole-cell proteome. (a) Representative flow cytometry dot plots and gel pixelation to illustrate procedure used to analyse cTregand eTregcell proteomes using mass spectrometry. (b) Area-proportional Venn diagrams illustrating the reproducibility of proteins identified in cTreg(left) or eTreg(right) cells from three independent experiments. WT cells were compared for this analysis and data were compiled using the intensity-based absolute quantification method. (c) A volcano plot illustrating differentially expressed proteins between eTregversus cTregcells in WT mice. (d) A volcano plot representing differentially expressed proteins between eTregcells fromNdfip1fl/flFoxp3-Cre or WT animals. (e) Network diagram of enriched GO terms with nodes representing GO annotations and edges connecting similar terms based on the GO hierarchy. The size of the nodes corresponds to the number of genes associated with the respective GO term and the colour of the nodes corresponds to the level of significance of the enrichment of the respective term in the data set (darker colour corresponds to a higher level of significance). Clusters of GO terms were manually analysed and annotated to identify broad functional similarity. Data are shown for YFP+eTregcells that were sorted from 9- to 12-week-old WT orNdfip1fl/flFoxp3-Cremale mice. Figure 6: Ndfip1 fl/fl Foxp3 -Cre eT reg cells have altered metabolic whole-cell proteome. ( a ) Representative flow cytometry dot plots and gel pixelation to illustrate procedure used to analyse cT reg and eT reg cell proteomes using mass spectrometry. ( b ) Area-proportional Venn diagrams illustrating the reproducibility of proteins identified in cT reg (left) or eT reg (right) cells from three independent experiments. WT cells were compared for this analysis and data were compiled using the intensity-based absolute quantification method. ( c ) A volcano plot illustrating differentially expressed proteins between eT reg versus cT reg cells in WT mice. ( d ) A volcano plot representing differentially expressed proteins between eT reg cells from Ndfip1 fl/fl Foxp3- Cre or WT animals. ( e ) Network diagram of enriched GO terms with nodes representing GO annotations and edges connecting similar terms based on the GO hierarchy. The size of the nodes corresponds to the number of genes associated with the respective GO term and the colour of the nodes corresponds to the level of significance of the enrichment of the respective term in the data set (darker colour corresponds to a higher level of significance). Clusters of GO terms were manually analysed and annotated to identify broad functional similarity. Data are shown for YFP + eT reg cells that were sorted from 9- to 12-week-old WT or Ndfip1 fl/fl Foxp3-Cre male mice. Full size image To characterize differential protein expression in Ndfip1-sufficient and -deficient T reg cells, we compared the ratio of protein abundance in eT reg :cT reg for each of the three experiments. This revealed widespread changes in the proteomes of Ndfip1-deficient T reg cells. Given that Ndfip1 deficiency drove changes predominantly in eT reg cells, we focussed our comparisons on the levels of proteins identified in WT and Ndfip1-deficient eT reg cells ( Supplementary Data 2 and Fig. 6d ). Our flow cytometric finding of increased GITR expression was supported by these T reg proteomes ( Supplementary Data 2 and Fig. 6d ). Surprisingly, proteins associated with increased mTORC1 activity were increased in Ndfip1-deficient eT reg cells. This included Lamtor1 ( Fig. 6d ), as well as the V-ATPase subunit d1 and Lamtor3, which are components of the v-ATPase-regulator complex that drives mTORC1 activation in cells [31] , [32] , [33] . We then performed network visualization of gene-ontology (GO) enrichment analysis for differentially regulated proteins in Ndfip1-sufficient and -deficient eT reg cells and identified clusters of nodes relating to metabolic processes that were significantly enriched ( Fig. 6e and Supplementary Data 2 ). Pathway analysis further supported changes in the metabolic state of Ndfip1-deficient eT reg cells and, more specifically, an increase in mTORC1 activity. Thus loss of Ndfip1 led to an altered proteomic profile indicative of altered metabolic activity. Ndfip1-deficient T reg cells have increased glycolysis Based on this proteomics profiling, we sought to analyse the metabolic capacity of Ndfip1-deficient T reg cells. To obtain sufficient cell numbers for metabolic testing, we used in vitro IL-2-expanded T reg cells. We evaluated the bioenergetics of these expanded WT and Ndfip1 fl/fl Foxp3- Cre T reg cells at ‘rest’ and also upon restimulation. We measured the extracellular acidification rate under glycolytic stress conditions ( Fig. 7a–d ) and oxygen consumption rate under mitochondrial stress conditions ( Fig. 7e–h ). Prior to stimulation, WT T reg cells had low basal rates of glycolysis, but rates increased when cells were stimulated ( Fig. 7a,b ). In Ndfip1-deficient T reg cells, the ‘resting’ glycolytic rate was only modestly increased over WT cells ( Fig. 7a,c ). However, restimulated Ndfip1-deficient T reg cells had a considerably increased glycolytic rate and glycolytic capacity compared to restimulated WT T reg cells ( Fig. 7b–d ). To assess mitochondrial function, we measured cell respiratory control, which is a general test of mitochondrial function in cells. Loss of Ndfip1 did not change the maximum respiratory capacity of T reg cells and caused a slight decrease in the spare respiratory capacity of T reg cells ( Fig. 7e–h ). Taken together, these data indicate that the loss of Ndfip1 drives a metabolic switch in activated T reg cells, promoting a more effector cell-like reliance on glycolysis to supply cellular energetic demands. 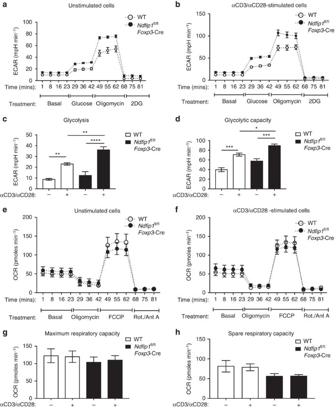Figure 7: Ndfip1-deficient Tregcells have a significantly increased rate of glycolysis. (a–h) YFP+Tregcells were sorted fromNdfip1+/+Foxp3-Cre WT orNdfip1fl/flFoxp3-Cremice, expanded in culture and then were left unstimulated or were restimulated before metabolic function was assessed. (a,b) Extracellular acidification rate (ECAR) was measured during a glycolysis stress test inaunstimulated or (b) stimulated Tregcells treated with drugs as indicated. (c) Rate of glycolysis is the difference in ECAR between post-glucose addition and baseline. (d) Glycolytic capacity is the difference between post-Oligomycin ECAR and baseline ECAR. (e,f) Oxygen consumption rate (OCR) changes during a mitochondrial function assessment test ineunstimulated or (f) stimulated WT orNdfip1fl/flFoxp3-Cre Tregcells treated with drugs as indicated. (g) Maximum respiratory capacity is the difference in OCR after addition of rotenone/Antimycin A versus after addition of fluoro-carbonyl cyanide phenylhydrazone (FCCP). (h) Spare respiratory capacity is the difference in increased OCR following addition of FCCP compared to baseline. Graphs show mean±s.e.m. (a–d) Representsn=4 mice (male or female, 7–12 weeks) per genotype in two independent experiments. Final Foxp3% afterin vitroexpansion was 74.45%±8.03 forNdfip1fl/flFoxp3-Cre versus 74.8±9.80 forNdfip1+/+Foxp3-Cre. (e–h) Representsn=6–8 mice (male and female, 7–12 weeks) in three experiments. Final Foxp3% was 88.1±2.08 forNdfip1fl/flFoxp3-Cre versus 86.43±1.94 forNdfip1+/+Foxp3-Cre.Pvalues were calculated by one-way ANOVA. *P<0.05, **P<0.01, ***P<0.001, ****P<0.0001. Figure 7: Ndfip1-deficient T reg cells have a significantly increased rate of glycolysis. ( a – h ) YFP + T reg cells were sorted from Ndfip1 +/+ Foxp3- Cre WT or Ndfip1 fl/fl Foxp3-Cre mice, expanded in culture and then were left unstimulated or were restimulated before metabolic function was assessed. ( a , b ) Extracellular acidification rate (ECAR) was measured during a glycolysis stress test in a unstimulated or ( b ) stimulated T reg cells treated with drugs as indicated. ( c ) Rate of glycolysis is the difference in ECAR between post-glucose addition and baseline. ( d ) Glycolytic capacity is the difference between post-Oligomycin ECAR and baseline ECAR. ( e , f ) Oxygen consumption rate (OCR) changes during a mitochondrial function assessment test in e unstimulated or ( f ) stimulated WT or Ndfip1 fl/fl Foxp3- Cre T reg cells treated with drugs as indicated. ( g ) Maximum respiratory capacity is the difference in OCR after addition of rotenone/Antimycin A versus after addition of fluoro-carbonyl cyanide phenylhydrazone (FCCP). ( h ) Spare respiratory capacity is the difference in increased OCR following addition of FCCP compared to baseline. Graphs show mean±s.e.m. ( a – d ) Represents n =4 mice (male or female, 7–12 weeks) per genotype in two independent experiments. Final Foxp3% after in vitro expansion was 74.45%±8.03 for Ndfip1 fl/fl Foxp3- Cre versus 74.8±9.80 for Ndfip1 +/+ Foxp3- Cre. ( e – h ) Represents n =6–8 mice (male and female, 7–12 weeks) in three experiments. Final Foxp3% was 88.1±2.08 for Ndfip1 fl/fl Foxp3- Cre versus 86.43±1.94 for Ndfip1 +/+ Foxp3- Cre. P values were calculated by one-way ANOVA. * P <0.05, ** P <0.01, *** P <0.001, **** P <0.0001. Full size image Ndfip1-deficient T reg cells have elevated mTORC1 activity Effector T cells utilize glycolysis while T reg cells are more dependent on oxidative phosphorylation as their main source of energy [34] , [35] , [36] , [37] , [38] . High glycolytic activity in T reg cells, as can occur when mTORC1 activity is increased, has been associated with T reg cell dysfunction [6] , [7] , [39] . To investigate whether mTORC1 activity was increased in Ndfip1-deficient T reg cells, we cultured WT and Ndfip1 fl/fl Foxp3- Cre T reg cells in vitro . We found that Ndfip1 fl/fl Foxp3- Cre T reg cells quickly outnumbered their WT counterparts ( Fig. 8a ), were increased in cell size ( Fig. 8b ) and proliferated more ( Fig. 8c ). This, together with observed increases in ICOS and GITR expression ( Fig. 8d,e ), suggested that this in vitro culture system recapitulates the phenotype of Ndfip1-deficient T reg cells in vivo . Given that ICOS can be driven by mTORC1 (ref. 39 ) activity, we examined other proteins in the mTORC1 pathway, including the amino acid transporter, CD98, and phosphorylated S6 (pS6). CD98 and pS6 ( Fig. 8f,g ) were both increased in Ndfip1 fl/fl Foxp3- Cre T reg cells. Coculture confirmed that these changes are not directly linked to IL-4 signalling ( Fig. 8h ). 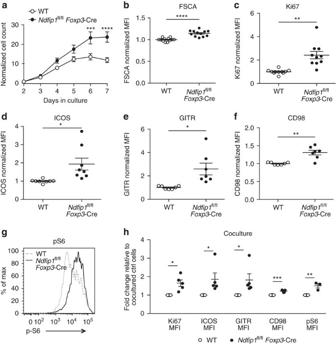Figure 8: Loss of Ndfip1 leads to elevated mTORC1 signalling and metabolic fitness in Tregcells. (a–h) Tregcells were sorted from congenically distinct CD45.1 WT or CD45.2Ndfip1fl/flFoxp3-Cre mice. Tregcells were expandedin vitro(a–g) individually or (h) in mixed cocultures. (a) Cell numbers in the cultures were analysed daily for 7 days. (b–f) After 7 days, cells were analysed by flow cytometry for cell size (forward scatter (FSC)), (b) Ki67 expression, (c) or their surface levels of: (d) ICOS, (e) CD98, and (f) GITR. (g) Cells were also restimulated at the end of the culture period and analysed for expression of pS6. (h) Cocultured WT andNdfip1fl/flFoxp3-Cre Tregcells were similarly examined for the expression of Ki67, ICOS, GITR, CD98 and pS6. Each dot represents an individual mouse. All experiments were performed on at least two independent occasions using age-matched male or female, aged 7–12 weeks, mice of each genotype.Pvalues were calculated by multiplet-tests. *P<0.05, **P<0.01, ***P<0.001, ****P<0.0001. Error bars indicate mean±s.e.m. Figure 8: Loss of Ndfip1 leads to elevated mTORC1 signalling and metabolic fitness in T reg cells. ( a – h ) T reg cells were sorted from congenically distinct CD45.1 WT or CD45.2 Ndfip1 fl/fl Foxp3- Cre mice. T reg cells were expanded in vitro ( a – g ) individually or ( h ) in mixed cocultures. ( a ) Cell numbers in the cultures were analysed daily for 7 days. ( b – f ) After 7 days, cells were analysed by flow cytometry for cell size (forward scatter (FSC)), ( b ) Ki67 expression, ( c ) or their surface levels of: ( d ) ICOS, ( e ) CD98, and ( f ) GITR. ( g ) Cells were also restimulated at the end of the culture period and analysed for expression of pS6. ( h ) Cocultured WT and Ndfip1 fl/fl Foxp3- Cre T reg cells were similarly examined for the expression of Ki67, ICOS, GITR, CD98 and pS6. Each dot represents an individual mouse. All experiments were performed on at least two independent occasions using age-matched male or female, aged 7–12 weeks, mice of each genotype. P values were calculated by multiple t -tests. * P <0.05, ** P <0.01, *** P <0.001, **** P <0.0001. Error bars indicate mean±s.e.m. Full size image Increased responsiveness to IL-2 could explain the fitness of Ndfip1-deficient T reg cells in this IL-2 expansion system. To test this, we sorted Ndfip1-sufficient and -deficient T reg cells and rested them overnight without cytokine or TCR stimulation. Upon brief IL-2 stimulation, we detected STAT5 phosphorylation (pSTAT5) by flow cytometry. pSTAT5 levels (mean fluorescence intensity) were similar between WT and Ndfip1-deficient T reg cells before and after IL-2 stimulation ( Supplementary Fig. 8 ). This is consistent with our recent report showing that both Ndfip1 and its homologue, Ndfip2, are required in T conv cells to drive the degradation of Jak1 and decrease STAT5 phosphorylation in response to IL-2 (ref. 40 ). Therefore, the increased metabolic activity of Ndfip1 fl/fl Foxp3-Cre + T reg cells is cell intrinsic and not just because of enhanced responsiveness to IL-2. Therapies using adoptively transferred T reg cells or that target T reg cell function are now being developed, making it essential to understand mechanisms that maintain T reg cell identity and how these pathways integrate with TCR activation and cellular metabolic processes. Our data identify Ndfip1, an activator of E3 ubiquitin ligases, as a new molecular target impacting T reg stability and function. We demonstrate that Ndfip1-deficient T reg cells are highly proliferative and concomitantly gain the capacity to produce the proinflammatory cytokine IL-4. Importantly, Ndfip1 deficiency can lead to the expansion of T reg cells and loss of Foxp3 in vivo . Both mTORC1 and mTORC2 play important functions in preventing T reg cells from adopting a glycolytic metabolic profile. mTORC1-mediated glycolytic activity in T reg cells is modulated by the serine–threonine phosphatase, PP2A, and by the autophagy proteins, Atg5 and Atg7 (refs 7 , 8 ). The lipid phosphatase, PTEN, inhibits mTORC2-mediated metabolic pathways in T reg cells to prevent T reg cell instability and maintain suppression of Th1 and Tfh effector T-cell functions [41] , [42] . Ndfip1-deficient T reg cells have increased protein levels of ICOS, CD98 and pS6, all indicators of high mTORC1 signalling. mTORC1 deletion in T reg cells leads to defects in efficiently synthesizing lipids from glucose and to defects in homeostatic proliferation in vivo [39] . Therefore, it is not surprising that Ndfip1-deficient T reg cells, with high mTORC1 signature, show greater homeostatic expansion in vivo , show greater metabolic fitness in vitro and in vivo and are more efficient at glycolysis. This altered glycolytic metabolism fuels dysfunction in vivo by driving the expansion of eT reg cells that are prone to produce IL-4 and lose Foxp3. We propose that T reg cells lacking Ndfip1 progress through a series of changes that is precipitated by increased proliferation of activated (CD44 + ) T reg cells and accompanied by the acquisition of IL-4 production. These changes are likely initiated in eT reg cells since Ndfip1 is inducibly expressed upon T-cell activation. The elevated glycolytic metabolism in these cells drives further expansion of IL-4-producing current and former T reg cells. Autocrine IL-4 signalling can then lead to loss of Foxp3. Supporting this, CD44 + Ndfip1-deficient T reg cells have increased methylation at the CNS2 region of the Foxp3 locus, indicating susceptibility towards instability. Ndfip1-deficient T H 2 cells are capable of driving tissue damage and inflammation as already described by our laboratory and others [12] , [14] , [40] , [43] . Loss of IL-4 did not affect the activation, proliferation and in vivo expansion of Ndfip1-deficient T reg cells leading us to conclude that the metabolic fitness in Ndfip1-deficient T reg cells precedes or is independent of the gain in T reg cell-intrinsic IL-4 production. Furthermore, IL-4-overexpressing transgenic mice have been described and have increased recruitment of different immune cell subsets into the skin but do not develop spontaneous dermatitis [44] as observed in Ndfip1 fl/fl Foxp3- Cre mice. Last, loss of the mTORC1 subunit, Raptor, in T reg cells does not lead to a cell-intrinsic increase in T reg cell IL-4 or other effector cytokines [39] , suggesting that cytokine regulation and metabolic regulation by Raptor in T reg cells may be two independent events [39] . An attractive hypothesis that warrants further future investigation is whether two parallel (but perhaps cross-talking) cellular pathways are regulated by Ndfip1: one which dampens mTORC1 activity and glycolysis in order to limit T reg cell activation and proliferation, and a second that limits T reg cell IL-4 production. These pathways, though independent, may cooperate to account for the severity of the inflammation observed in Ndfip1 fl/fl Foxp3- Cre mice. Ndfip1 is a known activator of Itch [40] , [45] , [46] . Mice bearing a T reg -specific deletion of Itch show some overlapping features with the Ndfip1 fl/fl Foxp3- Cre mice described here [15] : Itch-deficient T reg cells have an effector T reg cell phenotype, an increase in proliferation and intact suppression in traditional in vivo and in vitro suppression assays. Itch-deficient T reg cells are unstable as defined by their increased production of IL-4 but these T reg cells do not have defects in their ability to maintain Foxp3 expression in a lymphoreplete animal [15] . Future work will be needed to determine whether mTORC1 signalling is elevated in Itch-deficient T reg cells and whether this contributes to their dysfunction. Future studies on Itch and Ndfip1 will be of particular interest as therapies that activate or inhibit these pathways are being developed. If such therapeutic strategies can be used to regulate T reg cell functions, their use in the clinic could have broad potential. Mouse strains Ndfip1 fl/fl mice [47] were crossed to Foxp3-YFP- Cre reporter mice (Jackson Laboratory, stock# 016959 [17] ), also referred to as Foxp3- Cre, and bred for only one copy of the Cre gene to generate Ndfip1 fl/fl Foxp3- Cre male mice and Ndfip1 fl/fl Foxp3- Cre +/− female mice. WT control mice were: Ndfip1 +/+ Foxp3- Cre + male, and Ndfip1 +/+ Foxp3- Cre +/− female mice. We generated congenic CD45.1/CD45.2 control mice by crossing Ndfip1 +/+ Foxp3- Cre + mice to CD45.1 mice (Jackson Laboratory, Stock# 002014). CD45.1 and Rag1 −/− are maintained in house. Ndfip1 IL-4 DKO mice [25] , [26] are maintained in house. The gender and ages of mice used are indicated in each figure legend. Mice were maintained in a barrier facility at the Children’s Hospital of Philadelphia. All procedures were approved by the Institutional Care and Use Committee of the Children’s Hospital of Philadelphia. Genotyping primer sequences used were: Ndfip1 flox alleles ( Ndfip1 floxed forward 5′-TGAGGAAACAGACACACAATG-3′, Ndfip1 floxed reverse 5′-TGGAATGAACCTGAGGTCTCC-3′) [48] and Foxp3- Cre (Jackson Laboratory, stock# 016959, WT Forward: 5′-CCTAGCCCCTAGTTCCAACC-3′, WT Reverse: 5′-AAGGTTCCAGTGCTGTTGCT-3′, Mutant Forward: 5′-AGGATGTGAGGGACTACCTCCTGTA-3′, Mutant Reverse: 5′-TCCTTCACTCTGATTCTGGCAATTT-3′) [17] . Sequences for Il4 genotyping (Jackson Laboratory, stock# 002253) are: Il4 common 5′-GTGAGCAGATGACATGGGGC-3′; Il4 WT 5′-CTTCAAGCATGGAGTTTTCCC-3′ and Il4 mutant 5′-GCCGATTGTCTGTTGTGCCCAG-3′. Flow cytometry The following flow cytometric antibodies were purchased from Biolegend: CD4 (GK1.5), CD8α (53-6.7), CD44 (IM7), IL-17A (TC11-18H10.1), CD3ɛ (17A2), CD45.2 (104), CD45.1 (A20) GITR (YGITR765), ICOS (C398.4A), and PD-1 (RMP1-30), all used at 1:200 dilution. αYFP/GFP (A-21311) was purchased from Life Technologies and used at 1:400 dilution. Antibodies against IFNγ(XMG1.2) used at 1:300 and Ki67 (B56) used at 1:200 dilution were purchased from BD Biosciences. Biotinylated αphospho-S6 was purchased from Cell Signalling Technologies (D57.2.2E) and used at 1:150 dilution. The remaining antibodies for flow cytometry were purchased from eBioscience: CD25 (PC61.5), CD62L (MEL-14), and IL-10 (JES5-16E3) all used at 1:200 dilution; IL-4 (11B11) used at 1:100 dilution; and Foxp3-biotin (FJK-16s). Biotinylated αFoxp3 and αpS6 were used at 1:150 dilution and detected with fluorophore-conjugated streptavidin at 1:750 dilution (S32354 Invitrogen). Tissue processing and flow cytometry Serum was obtained by cardiac puncture immediately following CO 2 killing. Spleens and lymph nodes were harvested and mashed through 70 μM nylon filters using cold Hank’s Balanced Salt Solution (HBSS). Spleens were red blood cell (RBC) lysed using ammonium-chloride-potassium lysis buffer, washed, filtered again via a 70 μM filter and resuspended in cold HBSS for sorting or resuspended in complete DMEM (cDMEM) for either phorbol myristate acetate (PMA)/Ionomycin stimulation or direct flow cytometry. Lungs were flushed with cold phosphate-buffered saline (PBS) immediately after killing, minced in cDMEM medium containing 0.9 mg ml −1 of collagenase A (Sigma), 0.8 mg ml −1 of collagenase 1A (Sigma) and 20 μg ml −1 of DNase I (Sigma) and rotated for 1 h at room temperature. FCS was added at 15% v/v and the mixture was filtered through a 100 μM and then 40 μM filter before centrifugation. Lung pellets were RBC lysed using in-house-made ammonium-chloride-potassium lysis buffer, washed, resuspended in complete DMEM media and filtered through a 70 μm filter. The cells were then stimulated for 4 h in 5 ml round bottom polystyrene test tubes with PMA (30 ng ml −1 , Calbiochem), ionomycin (1 μM, Abcam) and Brefeldin A (1 μg ml −1 , Sigma) for intracellular cytokine staining or directly stained for flow cytometry. For flow cytometry, cells were washed in serum-free HBSS or PBS, stained with live/dead fixable blue dead cell stain (L-23105; Invitrogen, 1:60 dilution), Fc blocked (αCD16/32, 2.4G2; BD Biosciences, 1:25 dilution) and stained with the appropriate antibody mixtures. After staining 25 min at 4 °C, samples were washed in FACs buffer (1xPBS, 2.5% v/v FCS and 0.1%w/v Sodium azide) and then fixed overnight using the Foxp3 Fix/Perm Kit (00-5523-00, eBioscience). After washing with the provided Foxp3 kit perm buffer, intracellular staining was carried out for 1 h at 4 °C. Cells were washed again with perm buffer and resuspended for flow cytometry in FACs buffer. In Fig. 8 , expanded T reg cells, cultured as described below, were restimulated with mouse T-cell activator beads (Gibco, 11456D) at a 1:1 cell:bead ratio in complete DMEM medium for 4 h. Samples were immediately fixed at a final concentration of 2% PFA, permeabilized in 90% methanol and then stained for pS6 and surface markers together in Fc block. The same PFA fixation protocol was used for the pSTAT5 experiment. Samples were acquired on an LSRFortessa (BD Biosciences) and analysed using FlowJo version 9.8 (Flowjo LLC). Events analysed were singlets, (FSC-A × FSC-H, SSC-W × SSC-H), live (viability dye negative) and within the lymphocyte gate (FSC-A × SSC-A) ( Supplementary Fig. 9 ). Enzyme-linked immunosorbent assay (ELISA) Serum was isolated from 8- to 16-week-old male Ndfip1-sufficient and -deficient Foxp3-Cre + mice. The concentrations of Ig subclasses in mouse sera were determined using isotype-specific antibodies with a sandwich ELISA protocol. Monoclonal anti-mouse IgA-HRP, IgM-HRP, IgG1-HRP, IgG2C-HRP and IgE-HRP were purchased from SouthernBiotech. These were used in twofold serial dilutions starting at 10 ng ml −1 . Flat-bottom, 96-well plate (Nunc) was coated with capture antibody overnight at 1:250 dilution. Plates were blocked with 10% FCS in PBS buffer for 2 h and incubated with sample serum (1:20,000 for IgA, IgM and IgE and 1:40,000 for IgG1 and IgG2C) for 2 h at room temperature and detected with HRP-conjugated Ig subclass antibody (SouthernBiotech, 1:10,000 dilution) for 1 h at room temperature. Plates were developed with TMB substrate solution (eBioscience) and read at 450 nM using a Synergy HT Microplate Reader (BioTek). T-cell isolation YFP + CD4 + T reg cells were isolated from the spleen and lymph node, enriched for CD4 + T cells by negative selection using 5 μl per mouse of rat αmouse CD8α (2.43; Biolegend,) and 5 μl per mouse of rat αmouse I-A/I-E (M5/114.15.2; Biolegend) in 5–7.5 ml of complete DMEM medium and incubated for 30 min with end-over-end rotation at 4 °C. Cells were then washed and incubated with 1.5 ml of Biomag goat αrat IgG magnetic beads (Qiagen) for 10 min with end-over-end rotation at room temperature; unbound cells were collected using a Dynal magnet (Invitrogen). These enriched and untouched CD4 + T cells were then stained with antibodies against CD4, CD44, CD25 and CD62L all at 1:200 dilution. Cells were filtered through 35 μM filter cap polystyrene FACS tubes (BD Biosciences) and sorted under high speed on a MoFlow Astrios (Beckman Coulter) or a FACS Aria (BD Biosciences). Total T reg cells were sorted as CD4 + YFP + , cT reg cells as CD4 + YFP + CD62L high CD44 − and eT reg cells as CD4 + YFP + CD62L low CD44 + . Naive cells were identified as CD4 + CD62L high CD44 − CD25 − . Bisulfite sequencing Sodium bisulfite conversion, followed by PCR amplification and sequencing of individual clones, was used to determine the extent of CpG DNA methylation at the CNS2 and promoter regions of the Foxp3 gene. First, CD4 + YFP + CD62L low CD44 + eT reg cells were sorted from YFP + WT and Ndfip1 fl/fl Foxp3- Cre + mice. Naive CD4 + T cells were sorted from WT mice. Next, DNA was extracted using the Qiagen DNeasy Blood and Tissue Kit. Approximately 1 μg of DNA purified from CD4 + T reg cells was bisulfite converted via the following procedure [49] : the DNA was precipitated in ethanol, washed with 70% ethanol, and resuspended in 20 μl of Tris-EDTA buffer. This DNA was then denatured at 37 °C for 15 min using 0.3 M NaOH and then incubated at 55 °C for 16 h in a mixture containing 5.36 M Urea, 1.72 M sodium metabisulfite and 0.5 mM hydroquinone. The DNA was then desalted using the Wizard DNA clean-up system (Promega, A7170), desulfonated with 0.3 M NaOH, neutralized with 3 M ammonium acetate and precipitated with 100% ethanol. The CNS2 region of the Foxp3 gene was PCR amplified using the following primers: Foxp3 Intron Forward1 5′-GGGTTTTGGGATATTAATATATATAGTAAG-3′, Foxp3 Intron Reverse1 5′-CCACTATATTAACTTAACCCATATAACTAA-3′, Foxp3 Intron Forward2 5′-TTGAGTTTTTGTTATTATAGTATTTGAAGAT-3′, and Foxp3 Intron Reverse2 5′-ACTAAAAACCTAAAAAACTAAACTAACCAA-3′. The promoter region was amplified with the following primers: Foxp3 Promoter Forward1 5′-GTTTGGAGTAGAAGGAAGTTTTTGGAGAT-3′, Foxp3 Promoter Reverse1 5′-TATCTAAAAACCAACTACTCCACCTATCTA-3′, Foxp3 Promoter Forward2 5′-GGTTGTTTTTTATTTATATGGTAGGT-3′, and Foxp3 Promoter Reverse2 5′-CCAAAATCCTTACCTAAAATAACTA-3′. Following nested PCR, bands of appropriate sizes were gel purified and cloned into pGEM-T Easy vector (Promega, A1360). Single colonies were miniprepped with the QIAprep Spin Miniprep DNA Purification Kit (Qiagen, 27104) and sequenced with SP6 primer. Only sequences that were derived from fully converted alleles were used for methylation analysis. In vitro cell culture For the in vitro T reg cell suppression assay, sorted naive T conv CD45.1 + CD4 + CD62L high CD44 − CD25 − cells were stained with 2.5 μM carboxyfluorescein succinimidyl ester (CFSE) by incubating 400 μl of cells (10-20million cells per ml) in PBS with 400 μl of 5 mM CFSE in PBS solution for 3 min with continuous shaking. Next, 800 μl of FCS was added to the reaction mixture for 30 s at room temperature, followed by adding 10 ml of complete DMEM medium and spinning down in a centrifuge at 1300, r.p.m. for 5 min at 4–6 °C. The CFSE-labelled naive T conv cells were then resuspended to achieve 1.5 × 10 4 cells per 50 μl, and 50 μl of these cells were added to the appropriate wells of a 96-well plate. Sorted YFP + CD4 + CD45.2 + T reg cells were resuspended at 1.5 × 10 4 cells per 50 μl. A total of 50 μl of twofold serial dilutions of these T reg cells were added to the T conv cells in each well of the 96-well plate to achieve a final T reg :T conv ratio per well ranging from 0:1 to 1:32 (ref. 50 ). Next, irradiated bulk CD45.2 + splenocytes (2,500 rads, X-ray irradiator) were resuspended at 1.5 × 10 5 cells per 50 and 50 μl was added. Last, 50 μl of a 4 × solution containing αCD3 (145-2C11; Biolegend) and rhIL-2 were added to achieve a final concentration of 1 μg ml −1 soluble αCD3 and 50 U ml −1 IL-2 per well. The cells were cultured for 4 days for the suppression assay. For expanded T reg cultures, sorted YFP + CD4 + total T reg cells or CD4 + YFP + CD62L high CD44 − cT reg cells were resuspended at 1 × 10 6 cells per ml in media containing 2,000 U ml −1 IL-2 and stimulated at a 1:3 (cell:bead) ratio with mouse αCD3/αCD28 T-cell activator Dynabeads (Gibco, 11456D). After 48 h, cultures were counted and split daily with IL-2 media. Cells were assayed by flow cytometry after 6 or 7 days in cultures. Due to the 48-h activation, results from experiments where we started with sorted YFP + cT reg cells were virtually identical to those in which we started with sorted YFP + total T reg cells due to in vitro conversion of c T reg to e T reg cells. We therefore present all of that data pooled together. For analysis of RNA, expanded T reg cells were restimulated on day 7 of culture at a 1:1 ratio with αCD3/CD28 beads for the indicated periods. Supernatant was saved for ELISA and cells were harvested for quantitative PCR (qPCR). For cocultures, sorted WT and Ndfip-1 deficient T reg cells were mixed in a 1:1 ratio before being plated. For the in vitro stability assay using IL-2, IL-4 and αIL-2, WT or Ndfip1-deficient YFP + T reg cells were sorted from matched male or female donors. The T reg cells were cultured for 96 h on plate-bound 5 μg ml −1 αCD3/αCD28 and either 500 U ml −1 IL-2 or 20 ng ml −1 IL-4 with 20 ng ml −1 α-IL-2. All cultured cells, unless otherwise noted, were cultured at 10% CO 2 in complete T-cell medium, that is, DMEM (Mediatech) supplemented with 10% FCS (Atlanta Biologicals, premium FCS), 1% pen/strep (Invitrogen), 1% Glutamax (Invitrogen), 1% Minimum Essential Medium–non-essential amino acids (Invitrogen), 20 mM HEPES (Invitrogen), 1 mM Sodium Pyruvate and 0.12 mM betamercaptoethanol (Sigma) supplemented with recombinant human 50 U ml −1 IL-2 (originally obtained through the AIDS Research and Reference Reagent Program, Division of AIDS, National Institute of Allergy and Infectious Diseases, National Institutes of Health). Metabolic function assays YFP + CD44 − CD62L + T reg cells (cT reg cells ) or YFP + CD4 + T reg cells (total T reg cells ) were sorted from 7- to 12-week-old, age-matched male or female, congenically marked CD45.1 WT or CD45.2 Ndfip1 fl/fl Foxp3- Cre + (cKO) mice. After sorting, the WT or cKO T reg cells were expanded at a 1:3 (cell:bead) ratio with mouse αCD3/αCD28 beads for 7 days. On day 7, cells were harvested and resuspended at 5 × 10 6 cells per ml in appropriate Seahorse media. In all, 40 μl of cells were added to 140 μl of appropriate seahorse media or 140 μl of Seahorse media containing fresh mouse αCD3/αCD28 beads at a 1:1 (cell:bead) ratio. Cells were plated in XF96 cell culture microplates that were precoated with 25 μl of Cell tak reagent overnight according to the manufacturer’s instructions (Corning, 354240). For examining glycolysis, the glyco-stress test kit (Seahorse Bioscience) was used with additions of the following reagents to cells in glucose-free Seahorse media: 10 mM glucose, 2 μM oligomycin, and 50 mM 2-DG. To determine the rate of glycolysis, T reg cells were incubated in glucose-free medium and the increased extracellular acidification rate response upon stimulation of glycolysis by glucose and oligomycin was determined. Oligomycin inhibits mitochondrial ATP synthase (complex V) forcing glycolysis to compensate for the lack of ATP production in oxidative phosphorylation. Finally, 2-dexoglucose was added to inhibit glycolysis. For examining mitochondrial function, a mito-stress kit was used with additions of the following reagents to cells in appropriate Seahorse media: 2 μM Oligomycin, 1.5 μM fluoro-carbonyl cyanide phenylhydrazone (an uncoupler of respiration and oxidative ATP synthesis), and premixed 100 nM rotenone+1 μM antimycin A solution (Electron Transport Chain complex I and III inhibitors). Plates were run on an XF96 Seahorse assay instrument. Settings used were: calibration, equilibration, and baseline readings (loop three times). Before the baseline reading, and after each injection from a port, the following procedure was followed: mix, wait 3 min, and measure for 2 min with 3 min end loop [51] . Each reagent was added according to the volumes recommended by the Seahorse assay manufacturer. Quantitative PCR Samples for qPCR were lysed in Trizol (Ambion). RNA was extracted using chloroform and qPCR was performed as follows: 10 ng of cDNA was added to TaqMan Gene Expression Master Mix and TaqMan Gene Expression primer/probe mix specific for Ndfip1 (Applied Biosystems), according to the manufacturer’s protocol for a final reaction volume of 20 μl. qPCR was performed using an Applied Biosystems 7500 Real-Time PCR system. Each sample was assayed in triplicate along with the endogenous control (actin). Actb primer/probe (4352933E) was obtained from Applied Biosystems. Ndfip1 custom primers: Ndfip1 _F 5′-GCTCCTCCACCATACAGCAGC-3′; Ndfip1 _R 5′-CGATGGGGGCTTTGGAAATCCAG-3′, and Ndfip1 Taqman MGB probe: 5′-TTTGGAAATCCAGATTCATCTTTG-3′ were obtained from Applied Biosystems [40] . Relative mRNA expression of each gene of interest was calculated as 2 dCt , where dCt represents threshold cycle (Ct) of Actin beta minus Ct of gene of interest. Bone marrow chimeras Bone marrow from male Ndfip1 fl/fl Foxp3- Cre + (CD45.2 + ) or WT mice: Ndfip1 +/+ Foxp3- Cre + (CD45.1/CD45.2) or CD45.1 + mice was obtained by flushing femur and tibia with cold HBSS, RBC lysing and passing through a 70 μM filter. Cells were processed into a single-cell suspension, T cell depleted, resuspended in freezing media (90% FCS, 10% DMSO) and kept at −80 °C until used. Thawed cells were washed, counted, resuspended in sterile PBS, mixed 1:1 CD45.1:CD45.2 and injected intravenously into sublethally irradiated (400 rads, X-Ray irradiator) 6-week-old male Rag1 −/− recipients at 1 × 10 6 cells per mouse. Chimeras were kept on 5.3 ml of Trimethoprim/Sulfamethoxazole (200 mg sulfamethoxazole+40 mg trimethoprim per 5 ml) per 400 ml drinking water for the first 2 weeks after bone marrow transfer. Chimeras were analysed 8 weeks after transfer. Histology Skin (ear) and oesophagus were dissected and fixed in 10% neutral buffered formalin for at least 24 h. Lung were obtained after manual transcardial perfusion with 10 ml syringes containing PBS and fixed in 10% neutral buffered formalin. All organs were then embedded in paraffin, sectioned to 5 μm thickness and stained with Haematoxylin and Eosin. Images were obtained using a Leica DM4000B upright scope paired with a Spot RT/SE Slider camera (Children’s Hospital of Philadelphia Pathology Core). T-cell transfer colitis Naive CD4 + T cells from WT mice (CD45.1 + or CD45.1/CD45.2) and CD4 + YFP + T reg cells from CD45.2 + Ndfip1 fl/fl Foxp3- Cre and CD45.2 + Ndfip1 +/+ Foxp3- Cre male mice were isolated from the spleens and lymph nodes. Cells were resuspended in sterile PBS and congenic naive T cells were mixed at a 5:1 ratio with YFP + T reg cells. A total of 0.36 × 10 6 cells were injected intraperitoneally into 6–8-week-old Rag1 −/− mice. Mice were weighed weekly. Recipients of both genotypes were cohoused. At killing, mice were weighed, spleens were weighed and the spleens and lung were processed for flow cytometry as described above. A fraction of the total lung/spleen single-cell suspensions were stained with antibodies against CD4, CD45.1 and CD45.2 and sorted using a Moflow Astrios as described above for analysis of Ndfip1 mRNA in cells from Ndfip1 fl/fl Foxp3- Cre and Ndfip1 +/+ Foxp3- Cre donor T reg cells. Sorted cells were CD4 + CD45.2 + CD45.1 − YFP + (current T reg cells ) or CD4 + CD45.2 + CD45.1 − YFP − (former T reg cells) or CD4 + CD45.2 − CD45.1 + YFP- (T conv cells). Cells were stimulated for 5 h with plate-bound 5 μg ml −1 αCD3/CD28 at 3 × 10 5 cells per ml and harvested in Trizol for qPCR. The remaining fractions of total lung/spleen single-cell suspensions were either stained directly for flow cytometry or stimulated for 4 h with PMA/ionomycin in the presence of Brefeldin A to analyse cytokine production by flow cytometry. Preparation of lysates for whole-cell proteome analysis Ndfip1-sufficient and -deficient cT reg cells and eT reg cells were isolated and lysed using a lysis buffer containing 100 mM Tris-HCl, pH 8.0, 0.15 M NaCl, 5 mM EDTA, 1% NP-40, 0.5% Triton-X 100, protease inhibitor cocktail (Roche, 11697498001), 5 mM of 1,10-phenyanthroline ( o -PA), 5 mM N -ethymaleimide and 0.1 mM PR-619. In all, 10 μl of lysis buffer was used for every 10 × 10 6 cells. Protein was quantified by BCA (Pierce, 23227). Approximately 15 μg of lysate was mixed 1:1 with 4 × Laemmli sample buffer for whole proteome analysis. Samples were boiled and run ∼ 2 cm past the stacking gel in 10% Criterion precast Tris-HCL gels (Biorad). Gels were fixed overnight and stained briefly with Coomassie blue. Each lane of the Coomassie-stained gel was divided into 8–10 2 × 9 mm 2 ‘pixels,’ each cut into 1 mm 3 cubes [52] . They were destained with 50% Methanol/1.25% Acetic Acid, reduced with 5 mM dithiothreitol (Thermo) and alkylated with 40 mM iodoacetamide (Sigma). Gel pieces were then washed with 20 mM ammonium bicarbonate (Sigma) and dehydrated with acetonitrile (Fisher). Trypsin (5 ng μl −1 in 20 mM ammonium bicarbonate, Promega) was added to the gel pieces and proteolysis was allowed to proceed overnight at 37 °C. Peptides were extracted with 0.3% triflouroacetic acid (J.T. Baker), followed by 50% acetonitrile. Extracts were combined and the volume was reduced by vacuum centrifugation. Mass spectrometric analysis Tryptic digests were analysed by LC-MS/MS on a hybrid LTQ Orbitrap Elite mass spectrometer coupled with a Dionex Ultimate 3000 (Thermofisher Scientific San Jose, CA). Peptides were separated by reverse phase (RP) HPLC on a nanocapillary column, 75 μm id × 30 cm Reprosil-pur 1.9 μM (Dr Maisch, Germany). Mobile phase A consisted of 0.1% formic acid (Thermo) and mobile phase B of 0.1% formic in acetonitrile. Peptides were eluted into the mass spectrometer at 300 nl min −1 with each RP-LC run comprising a 90 min gradient from 3% to 45% B in 90 min. The mass spectrometer was set to repetitively scan m / z from 300 to 1,800 ( R =240,000 for LTQ-Orbitrap Elite) followed by data-dependent MS/MS scans on the 20 most abundant ions, with a minimum signal of 1,500, dynamic exclusion with a repeat count of 1, repeat duration of 30 s, exclusion size of 5,000 and duration of 60 s, isolation width of 2.0, normalized collision energy of 33 and waveform injection and dynamic exclusion enabled. Fourier transform MS full-scan AGC target value was 1e6, while MSn AGC was 1e4. Fourier transform MS full-scan maximum fill time was 10 ms, while ion trap MSn fill time was 100 ms; microscans were set at one. FT preview mode; charge state screening and monoisotopic precursor selection were all enabled with rejection of unassigned and 1+ charge states. Proteomic data analysis Proteomic data were analysed using Maxquant version 1.5.0.30 searching against the Uniprot complete mouse reference proteome, including isoforms, (updated 19 September 2013) and common laboratory contaminants. A minimum peptide length of six amino acids and a peptide and protein false discovery of 1% was required. The three biological replicates for Ndfip1-sufficient and -deficient eT reg cells and cT reg cells were analysed together, with match between runs and requantify turned on. Label-free quantification via intensity-based absolute quantification was calculated in MaxQuant. Quantification data were normalized by the mean quantification value of identified proteins in each replicate and log2 transformed. Comparisons of protein hits from WT or Ndfip1-deficient eT reg or cT reg cells were calculated by log2 fold changes and evaluated for significance using a one-sample t -test. Area-proportional Venn diagrams were generated with eulerAPE version 3.0 ( http://www.eulerdiagrams.org/eulerAPE/ ) [53] . The GO analysis and corresponding network diagram in Fig. 6e was generated with the BiNGO application [54] in Cytoscape [55] . The differentially regulated proteins identified in WT vs cKO eT reg comparisons were compared against the Mus musculus GO Biological Process annotation using a hypergeometric significance test with Benjamini–Hochberg false-discovery rate correction. A threshold of adjusted P value of <0.01 was required for enrichment. Statistical analysis Data were graphed and analysed for statistical significance in Prism version 6 or version 7 (Graphpad Software, Inc) or Excel (Microsoft). The heatmap in Fig. 5 was generated in prism 7. The following statistical tests were used as appropriate and as noted in the figure legends: t -test, one-way analysis of variance (ANOVA), two-way ANOVA, and repeated-measures ANOVA. All data are shown as average±s.e.m., with a cutoff of P <0.05 for statistical significance: * P <0.05, ** P <0.01, *** P <0.001, **** P <0.0001. Data availability All data generated or analysed during this study are included in this published article (and its Supplementary Information files). The mass spectrometric proteomics data have been deposited to the ProteomeXchange Consortium via the PRIDE [56] partner repository with the data set identifier PXD006251. How to cite this article: Layman, A. A. K. et al . Ndfip1 restricts mTORC1 signalling and glycolysis in regulatory T cells to prevent autoinflammatory disease. Nat. Commun. 8, 15677 doi: 10.1038/ncomms15677 (2017). Publisher’s note: Springer Nature remains neutral with regard to jurisdictional claims in published maps and institutional affiliations.